Two nested developmental waves demarcate a compartment boundary in the mouse lung The lung is a branched tubular network with two distinct compartments—the proximal conducting airways and the peripheral gas exchange region—separated by a discrete boundary termed the bronchoalveolar duct junction (BADJ). Here we image the developing mouse lung in three-dimensions (3D) and show that two nested developmental waves demarcate the BADJ under the control of a global hormonal signal. A first wave of branching morphogenesis progresses throughout embryonic development, generating branches for both compartments. A second wave of conducting airway differentiation follows the first wave but terminates earlier, specifying the proximal compartment and setting the BADJ. The second wave is terminated by a glucocorticoid signalling: premature activation or loss of glucocorticoid signalling causes a proximal or distal shift, respectively, in BADJ location. The results demonstrate a new mechanism of boundary formation in complex, 3D organs and provide new insights into glucocorticoid therapies for lung defects in premature birth. Physiological processes occur sequentially in discrete compartments of mammalian organs, such as digestion and absorption along the digestive tract, and filtration, absorption and secretion in the kidney. Compartment boundaries separate cells of different types and may constitute a unique environment for cell signalling. The mammalian lung is a tree-like structure consisting of two compartments: the conducting airways, which filter inhaled air and allow its passage into the distal lung by convection, and the gas exchange region, which undergoes structural specialization into alveoli that drastically increases surface area to facilitate the diffusion of oxygen and carbon dioxide. Both compartments consist of morphologically and molecularly distinct cell types required for their respective functions, including ciliated cells and Clara cells in the conducting airways and alveolar type I and type II cells in the gas exchange region [1] . Classic electron and light microscopy studies in multiple species have identified a discrete junction between these two epithelial compartments termed the bronchoalveolar duct junction (BADJ), which is characterized by an abrupt transition in cell type and morphology [2] , [3] , [4] , [5] . Recent studies have highlighted the importance of the BADJ as the niche for bronchoalveolar stem cells (BASCs) that express markers of both compartments and are potentially responsible for certain types of lung repair and lung cancer [6] , [7] , [8] . In relatively simpler systems with limited number of compartment boundaries, it is well established that compartment boundaries form in response to a gradient of diffusible proteins (morphogen gradient) or a combination of a morphogen gradient and an oscillating signal, and can be further refined through differential cell adhesion [9] , [10] , [11] , [12] . For example, classic studies show that the anterior and posterior compartments in a Drosophila embryo are marked by restricted expression of Hunchback in the anterior compartment, and that this compartment boundary results from localized production of Bicoid at the anterior pole, which diffuses posteriorly to form a concentration gradient and exceeds a threshold only in the anterior compartment to activate Hunchback expression [13] . In contrast, little is known about when and how compartment boundaries form in complex mammalian organs. The BADJ along the proximal–distal axis of the respiratory tree is analogous to the aforementioned compartment boundary along the anterior–posterior axis in the Drosophila embryo. However, the BADJ has several unique features. First, rather than a single compartment boundary, the BADJ forms at hundreds of locations throughout a respiratory tree and formation of these BADJs requires some level of coordination so that each air passage leads to a properly sized gas exchange compartment. Second, the respiratory tree is a 3D, hierarchical tubular network; therefore, the signal specifying the BADJ needs to operate within such a spatial complexity. Third, unlike boundary formation in preformed syncytial Drosophila embryos, BADJ formation occurs in the context of an intricate branching morphogenesis process that starts after the left and right lung buds emerge from the embryonic foregut [1] . Although a branch lineage has been determined for the airways formed during the first five of nine (E11–E19) days of embryonic lung development in mice [14] , it is unclear how late lung development proceeds, and how the BADJ and gas exchange region relate to the branch lineage. Recent lineage tracing studies suggest that the developing lung has multipotent epithelial progenitors that give rise to cells in the conducting airway and gas exchange compartments depending on developmental stage [15] . However, it is unclear how regulation of the multipotent epithelial progenitors is integrated with branching morphogenesis and BADJ formation. Given these unique features of the BADJ, it is unknown whether a spatial signal similar to the morphogen gradient in the Drosophila embryo is used to establish the hundreds of BADJs within the complex 3D respiratory tree. Using 3D fluorescence imaging, we molecularly defined the BADJ in 3D and traced the developmental history of the entire respiratory tree. We show that the two compartments are built in two waves—a first wave of branching morphogenesis followed by a second wave of conducting airway differentiation—and that the boundary between the two compartments, the BADJ, is specified temporally by a global hormone that terminates the second wave and promotes the formation of the gas exchange compartment. Therefore, two nested developmental waves set a compartment boundary under the control of a temporal signal. 3D definition of the BADJ in the mature lung The BADJ, historically demarcated by histological and functional criteria, is not well defined in the context of the 3D respiratory tree. Therefore, we developed multicolour immunofluorescence whole-mount staining and imaging methods to visualize the hundreds of BADJs in the entire lung at both macroscopic (whole lung) and microscopic (single cell) levels. Since no known gene is expressed only at the BADJ, we visualized the BADJ by staining for the complete conducting airways, similar to how the compartment boundary was marked by Hunchback expression in the anterior Drosophila embryos. We chose SRY-box-containing gene 2 (SOX2), a transcription factor expressed by cells in the conducting airways, instead of markers of differentiated conducting airway cells, such as Clara cell secretory protein (CCSP), because SOX2 is expressed early in development and is necessary and sufficient for conducting airway cell maturation [16] , [17] , [18] , [19] , [20] , and because CCSP is limited to a subpopulation of conducting airway cells (Clara cells) and to the mature lung, and CCSP lineage-positive cells have been identified in both epithelial compartments [7] , [21] , [22] . When we stained mature lungs for SOX2, all conducting airways were labelled continuously from the trachea ( Fig. 1a ), and the distal boundary of SOX2 staining coincided with those of CCSP and smooth muscle actin (SMA), a marker for smooth muscles surrounding the conducting airways. 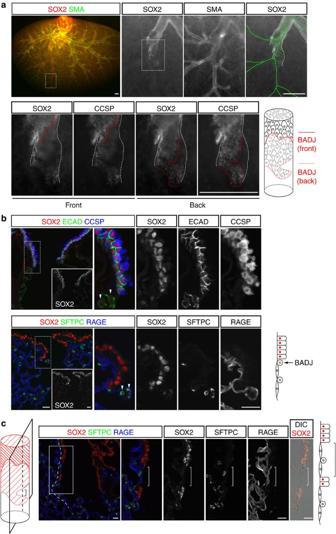Figure 1: 3D definition of the BADJ in the mature mouse lung. (a) Stereomicroscope images of a whole-mount immunostained cranial lung lobe from a 4-week-old mouse. SMA, smooth muscle actin; CCSP, Clara cell secretary protein. The boxed areas are enlarged in subsequent images. The conducting airways marked by SOX2 expression are traced with white dashed lines, and the BADJs, marked by the distal boundaries of SOX2 and CCSP expression domains, on the front and back sides of the tube are traced with solid and dashed red lines, respectively. The airway smooth muscles are traced with green dashed lines and the vascular smooth muscles are traced with solid green lines. The diagram illustrates significant irregularity in the shape of the BADJ around the perimeter of a terminal bronchiole. Conducting airway cells in the front (black) and back (grey) sides of the tube and the associated BADJs (solid and dashed red lines) are drawn. Scale: 250 μm. (b) Confocal images of immunostained sections of a 4-week-old mouse lung. ECAD, E-Cadherin; SFTPC, surfactant protein C; RAGE, receptor for advanced glycosylation of end products. Insets, SOX2 staining only. The boxed areas are enlarged in subsequent images. Some BADJs harbour 1~2 cells (arrowheads) with low level of SOX2 expression that also express SFTPC and may represent the BASCs. The diagram illustrates the difference in morphology and arrangement between cells in the conducting airways (filled red nuclei) and gas exchange region (black nuclei). Cells with open red nuclei represent the BASCs at the BADJ. Scale: 20 μm. (c) Confocal images of an immunostained section of a 4-week-old mouse lung showing that, depending on the local shape of the BADJ and the section plane (left diagram, the conducting airway in red), a conducting airway that is continuous in 3D can appear interrupted by alveolar type I and type II cells (brackets) on section (right diagram, seebfor symbol definition). One side of the tube is diagrammed and traced with long dashed lines, and the boxed area is enlarged in subsequent images. DIC, differential interference contrast. Scale: 20 μm. Figure 1: 3D definition of the BADJ in the mature mouse lung. ( a ) Stereomicroscope images of a whole-mount immunostained cranial lung lobe from a 4-week-old mouse. SMA, smooth muscle actin; CCSP, Clara cell secretary protein. The boxed areas are enlarged in subsequent images. The conducting airways marked by SOX2 expression are traced with white dashed lines, and the BADJs, marked by the distal boundaries of SOX2 and CCSP expression domains, on the front and back sides of the tube are traced with solid and dashed red lines, respectively. The airway smooth muscles are traced with green dashed lines and the vascular smooth muscles are traced with solid green lines. The diagram illustrates significant irregularity in the shape of the BADJ around the perimeter of a terminal bronchiole. Conducting airway cells in the front (black) and back (grey) sides of the tube and the associated BADJs (solid and dashed red lines) are drawn. Scale: 250 μm. ( b ) Confocal images of immunostained sections of a 4-week-old mouse lung. ECAD, E-Cadherin; SFTPC, surfactant protein C; RAGE, receptor for advanced glycosylation of end products. Insets, SOX2 staining only. The boxed areas are enlarged in subsequent images. Some BADJs harbour 1~2 cells (arrowheads) with low level of SOX2 expression that also express SFTPC and may represent the BASCs. The diagram illustrates the difference in morphology and arrangement between cells in the conducting airways (filled red nuclei) and gas exchange region (black nuclei). Cells with open red nuclei represent the BASCs at the BADJ. Scale: 20 μm. ( c ) Confocal images of an immunostained section of a 4-week-old mouse lung showing that, depending on the local shape of the BADJ and the section plane (left diagram, the conducting airway in red), a conducting airway that is continuous in 3D can appear interrupted by alveolar type I and type II cells (brackets) on section (right diagram, see b for symbol definition). One side of the tube is diagrammed and traced with long dashed lines, and the boxed area is enlarged in subsequent images. DIC, differential interference contrast. Scale: 20 μm. Full size image This SOX2-staining pattern ( Fig. 1a ) and our subsequent cellular analysis ( Fig. 1b ) allowed us to define the BADJ as the distal boundary of the SOX2 expression domain and to visualize the 3D morphology of the BADJ in the whole lung. SOX2-positive epithelial cells formed a continuous sheet from the trachea, stopping abruptly at the BADJ with no isolated SOX2-positive cells in the gas exchange region. However, the shape of the BADJ is highly irregular around the perimeter of individual terminal bronchioles—the most distal branches of the conducting airways—such that a patch of SOX2-positive cells frequently protruded further distally than the rest of the conducting airway with both convex and concave borders ( Fig. 1 ), forming peninsulas (but never islands) of SOX2-positive cells. This irregular shape was not apparent in prior studies of sagittal sections [23] and may contribute to the existence of the respiratory bronchiole—a hybrid lung tube with properties of both the conducting airway and gas exchange region that appears on sections as an air-conducting tube with its wall interrupted by pouches of alveoli [3] , [4] , [24] . Depending on the local shape of the BADJ and the section plane, a conducting airway continuous in 3D could appear interrupted by alveolar cells on sections ( Fig. 1c ), and a single conducting airway appeared as either a terminal bronchiole or a respiratory bronchiole on adjacent sections ( Supplementary Fig. 1a ). The molecular definition of the BADJ as the distal boundary of the SOX2 expression domain matched the classic cellular and morphological definitions of the BADJ as the boundary between cells in the conducting airways and gas exchange region. Clara cells, ciliated cells and neuroendocrine cells, but not basal cells, were found at the BADJ ( Fig. 1 and Supplementary Fig. 1b–d ), supporting that SOX2 expression marks a domain of the respiratory tree within which all four cell types of the conducting airway reside. Conversely, SOX2 was not expressed by alveolar type I cells marked by glycoprotein 38 (GP38) and receptor for advanced glycosylation of end products (RAGE) and type II cells marked by SFTPC (Fig. 1b and Supplementary Fig. 1e,f ); in addition, the compact cell arrangement of the conducting airway stopped at the boundary of the SOX2 expression domain, as shown by E-cadherin (ECAD, an epithelial cell junction marker) staining and bright-field imaging (Fig. 1b,c and Supplementary Fig. 1a ). We also examined SOX2 expression in the potential lung stem cells (the BASCs) and observed several low-SOX2-expressing cells at the BADJ that were double-positive for CCSP and SFTPC ( Fig. 1 and Supplementary Fig. 1g ) and therefore were the BASCs [6] . Owing to their low frequency, the BASCs were not included in subsequent analyses. A first wave generates both compartments Next, we examined the developmental origin of the BADJs by following SOX2 expression during lung development. To visualize and compare the 3D structures of developing lungs whose sizes change by one order of magnitude, we used a 3D microscopic technique, optical projection tomography (OPT) [25] . We imaged whole lungs harvested throughout embryonic development (E10 through E19) and immunostained for three potentially informative markers: ECAD, an epithelial marker; SOX2, a marker for the conducting airways in the mature lung; and SRY-box-containing gene 9 (SOX9), a marker associated with the distal lung epithelium undergoing branching morphogenesis in early development [26] , [27] , [28] . Our 3D images ( Fig. 2a ) allowed us to construct a complete developmental series of the entire respiratory tree, including the conducting airways and gas exchange region as well as the BADJs, and examine how the proximal–distal (SOX2–SOX9) patterning in the early developing lung was transformed into the two compartments in the mature lung. 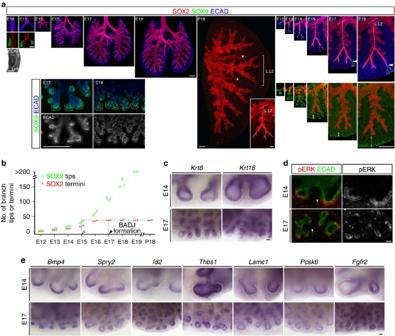Figure 2: A first wave generates both epithelial compartments. (a) OPT images of whole-mount immunostained lungs. All whole embryonic lungs and the P18 left lobe are shown to the same scale (scale: 500 μm) with the exception of the E10 foregut and E11 lung, which are shown at a higher magnification (Scale: 100 μm). In a side view of the E10 foregut, the nascent left lung bud (left) is outlined with a dashed line. The L.L2 branch lineages14are traced with dashed lines and shown as inset for the P18 lung and separately for the embryonic lungs (right panels, scale: 500 μm). Double-sided arrows indicate that the gap between the distal boundaries of the SOX2 and SOX9 expression domains widens after E17. Owing to variation in the branch lineage14, BADJ formation (closed arrowheads) are inferred by counting branches (b) and from lineage tracing experiments. Asterisks indicate that background staining from blood vessels only present in older postnatal lungs. Lower left panels (scale: 100 μm): projection of confocal images of immunostained E17 and E19 lung lobe edges for a high-resolution view of SOX9-positive branch tips (dashed line). (b) Quantification of the number of SOX9-positive branch tips (green circle) and SOX2-positive branch termini (red cross) of the planar bifurcation of L.L1 through L.L6 branch lineages14. The number of SOX2-positive termini plateaus at E17 (closed arrowhead). The number of SOX9-positive tips reaches the maximal number of SOX2-positive termini at E15 (open arrowhead). (c,e) Whole-mountin situhybridization of lungs at E14 (early branches) and E17 (late branches) for markers of simple epithelium (Krt8,Krt18(c)) and branching-related genes identified in anin silicoscreen of Eurexpress69(e). Branch tips are outlined with dashed lines. Scale: 20 μm. (d) Confocal images of whole-mount immunostained lungs at E14 (early branches) and E17 (late branches). pERK, phosphorylated extracellular signal-related kinase. pERK-positive branch tips are outlined with dashed lines. Cells in the vasculature are also pERK-positive (arrowheads). Scale: 20 μm. Figure 2: A first wave generates both epithelial compartments. ( a ) OPT images of whole-mount immunostained lungs. All whole embryonic lungs and the P18 left lobe are shown to the same scale (scale: 500 μm) with the exception of the E10 foregut and E11 lung, which are shown at a higher magnification (Scale: 100 μm). In a side view of the E10 foregut, the nascent left lung bud (left) is outlined with a dashed line. The L.L2 branch lineages [14] are traced with dashed lines and shown as inset for the P18 lung and separately for the embryonic lungs (right panels, scale: 500 μm). Double-sided arrows indicate that the gap between the distal boundaries of the SOX2 and SOX9 expression domains widens after E17. Owing to variation in the branch lineage [14] , BADJ formation (closed arrowheads) are inferred by counting branches ( b ) and from lineage tracing experiments. Asterisks indicate that background staining from blood vessels only present in older postnatal lungs. Lower left panels (scale: 100 μm): projection of confocal images of immunostained E17 and E19 lung lobe edges for a high-resolution view of SOX9-positive branch tips (dashed line). ( b ) Quantification of the number of SOX9-positive branch tips (green circle) and SOX2-positive branch termini (red cross) of the planar bifurcation of L.L1 through L.L6 branch lineages [14] . The number of SOX2-positive termini plateaus at E17 (closed arrowhead). The number of SOX9-positive tips reaches the maximal number of SOX2-positive termini at E15 (open arrowhead). ( c , e ) Whole-mount in situ hybridization of lungs at E14 (early branches) and E17 (late branches) for markers of simple epithelium ( Krt8 , Krt18 ( c )) and branching-related genes identified in an in silico screen of Eurexpress [69] ( e ). Branch tips are outlined with dashed lines. Scale: 20 μm. ( d ) Confocal images of whole-mount immunostained lungs at E14 (early branches) and E17 (late branches). pERK, phosphorylated extracellular signal-related kinase. pERK-positive branch tips are outlined with dashed lines. Cells in the vasculature are also pERK-positive (arrowheads). Scale: 20 μm. Full size image As early as lung specification at E10, SOX9 expression started in the nascent lung buds in the anterior foregut ( Fig. 2a ). Consistent with previous reports [26] , [27] , [28] , SOX9 was invariably associated with the distal epithelium generating new branches early in development (before E15). Surprisingly, we found that this branching process continued throughout embryonic development even during the canalicular and saccular stages of lung development (E18 and E19 (ref. 29 , Fig. 2a,b and Supplementary Fig. 2a ). New branches at early (E14) and late (E17) stages were formed by a similar process: both were simple epithelia ( Fig. 2c ); activated the ERK (extracellular signal-regulated kinase) signalling ( Fig. 2d ) and branching-related genes, such as Fgfr2 , Bmp4 , Spry2 , Id2 , Thbs1 , Lamc1 and Pcsk6 ( Fig. 2e and Supplementary Fig. 2b,c ); recruited smooth muscles ( Supplementary Fig. 2d ); and co-aligned with the vasculature ( Supplementary Fig. 2e ). As described in detail below, among all the branches generated via this continuous branching process, some became the conducting airways while others became the gas exchange region. Therefore, despite the grossly different structures and functions of the two compartments, both are formed by a similar and continuous process of branching morphogenesis, which we refer to as the first developmental wave—the branching morphogenesis wave (the SOX9 wave), by analogy to the centrifugal expansion of a physical wave from a point source (the equivalent of the trachea). A second wave establishes the BADJs New branches left behind by the first wave stopped expressing SOX9 and activated SOX2 in early development (before E15, Fig. 2a ). SOX2 expression persisted and marked the conducting airways in the mature lung and appeared to be the earliest event of conducting airway differentiation; this, together with the role of Sox2 in promoting mature conducting airway cells [16] , [17] , [18] , [19] , [20] , led us to name this centrifugal expansion of SOX2 expression the second developmental wave—the conducting airway differentiation wave (the SOX2 wave). While the expansions of SOX9 and SOX2 expression domains were coupled in early development, such a coupling was interrupted at E17—progression of the SOX2 wave was terminated while the SOX9 wave was still progressing, generating a large gap between the two-wave fronts ( Fig. 2a ). After E17, newly generated branches did not express SOX2 or contribute to the conducting airways, which grew with an increase only in length and diameter but not in branch number. Such independent progression of the two waves was more clearly demonstrated by counting branch tips and termini at the front of the SOX9 and SOX2 waves, respectively ( Fig. 2b ). The number of SOX9-positive tips increased exponentially throughout embryonic development, reflecting the continuous progression of the branching morphogenesis wave, whereas the number of SOX2-positive termini increased early in development but plateaued at E17, reflecting the completion of new conducting airways and therefore the formation of the BADJ. This divergence of the number of SOX2 termini from that of SOX9 tips ( Fig. 2b ) is unexpected from simple extrapolation of the known proximal–distal patterning of early developing lungs to late developmental stages, which will predict a parallel increase in the numbers of SOX2 termini and SOX9 tips throughout development. The uncoupling between the two waves was supported by Sox9 CreER lineage tracing experiments showing that SOX9-expressing cells in the first wave contributed significantly to the second wave before, but not after, E15 ( Supplementary Fig. 3a,b ), a finding consistent with previous Id2 CreER lineage tracing results [15] . These data, together with the branch counting results showing that the number of SOX9-positive tips reached the maximal number of SOX2-positive termini at E15 ( Fig. 2b ), suggested that cells near the BADJ are present at the very distal region of branch tips at E15, and that during the next 2 days some daughter cells become branch stalks, lose SOX9 expression and activate SOX2 at the BADJ at E17. The developmental origin of the BADJ was corroborated by Sox2 CreER lineage tracing experiments showing that the second wave marker SOX2 prospectively marked the conducting airways and the BADJ, but not the gas exchange region, in the mature lung. As predicted in our model ( Fig. 3b ), when recombination was induced early in development (before E17) while the SOX2 wave was still progressing, the lineage-labelled cells were distributed in a gradient within the conducting airways in the mature lung with high cell density proximally and low cell density distally ( Fig. 3 and Supplementary Fig. 3c ). When recombination was induced late in development, at or after the time of BADJ formation (E17), the lineage-labelled cells were evenly distributed along the proximal–distal axis of the mature conducting airways. Furthermore, the distal boundary of lineage-labelled cells in the mature lung progressed uniformly along all ramifications of the conducting airways as a function of the time of the lineage-labelling ( Fig. 3 and Supplementary Fig. 3c ). Importantly, the BADJs in the mature lung were lineage-labelled when recombination was induced at or after E17 ( Fig. 3d and Supplementary Fig. 3d ), the same time predicted for BADJ formation based on our quantitative analysis of fixed lungs ( Fig. 2a,b ). The Sox2 CreER lineage tracing experiments also excluded the possible model where the conducting airways and the BADJ form simply as a result of proliferation and distal expansion of existing SOX2-positive cells without conversion of newly formed branches to the conducting airways, which predicts that the BADJ should be lineage-labelled much earlier than observed. 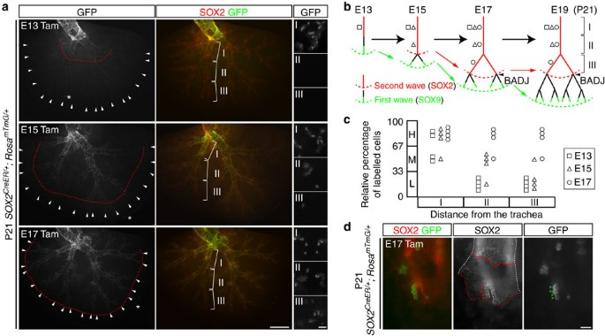Figure 3: A second wave establishes the BADJ. (a) Stereomicroscope images of whole-mount immunostained cranial lobes. Lineage-labelling is induced with tamoxifen (Tam) at indicated embryonic days. The distal boundaries of GFP-expressing cells (lineage markers) and those of SOX2-expressing cells (BADJs) are marked by red dashed lines and white arrowheads, respectively. The conducting airways along the RCr.L1 lineage14are divided into three regions of equal length (I, II and III) and representative high-magnification images of GFP-expressing cells in each region are shown (right column). No alveolar cells are lineage-labelled. Asterisks indicate nonspecific staining because of antibody trapping. Scale: 1,000 μm (left and middle columns) and 20 μm (right column). (b) Two-wave model superimposed by theSox2CreERlineage tracing schematics. Branches are generated by the first wave of branching morphogenesis (green dashed curves connected with green arrows) with SOX9-positive tips (green). Branches generated early (before E15), but not late (after E17), activate SOX2 expression (red) and constitute the second wave of conducting airway differentiation (red dashed curves connected with red arrows). The BADJ forms (arrowhead) when the second wave terminates at E17. The most proximal portions of the respiratory tree are SOX2-positive branched structures at E13 and are shown as red vertical lines for simplicity (square bracket I). The predicted distributions ofSox2CreERlineage cells labelled at E13 (square), E15 (triangle) and E17 (circle) are shown along the respiratory trees. The three portions (I, II and III) in the mature (P21) airways (a) are illustrated on the schematics of the E19 lung. (c) Percentage of labelled cells at indicated positions (I, II and III) relative to those in the extrapulmonary bronchus of the same lung that have been lineage-labelled at E13 (square), E15 (triangle) and E17 (circle). H: high (67–100%), M: medium (33–67%), L: low (0–33%). (d) Stereomicroscope images of a whole-mount immunostained P21 lung lineage-labelled at E17. The conducting airways are traced with white dashed lines, and the BADJs at the front and back of the branch are marked with solid and dashed red lines, respectively. The lineage-labelled cells at the BADJ are marked with horizontal carets. Scale: 20 μm. Figure 3: A second wave establishes the BADJ. ( a ) Stereomicroscope images of whole-mount immunostained cranial lobes. Lineage-labelling is induced with tamoxifen (Tam) at indicated embryonic days. The distal boundaries of GFP-expressing cells (lineage markers) and those of SOX2-expressing cells (BADJs) are marked by red dashed lines and white arrowheads, respectively. The conducting airways along the RCr.L1 lineage [14] are divided into three regions of equal length (I, II and III) and representative high-magnification images of GFP-expressing cells in each region are shown (right column). No alveolar cells are lineage-labelled. Asterisks indicate nonspecific staining because of antibody trapping. Scale: 1,000 μm (left and middle columns) and 20 μm (right column). ( b ) Two-wave model superimposed by the Sox2 CreER lineage tracing schematics. Branches are generated by the first wave of branching morphogenesis (green dashed curves connected with green arrows) with SOX9-positive tips (green). Branches generated early (before E15), but not late (after E17), activate SOX2 expression (red) and constitute the second wave of conducting airway differentiation (red dashed curves connected with red arrows). The BADJ forms (arrowhead) when the second wave terminates at E17. The most proximal portions of the respiratory tree are SOX2-positive branched structures at E13 and are shown as red vertical lines for simplicity (square bracket I). The predicted distributions of Sox2 CreER lineage cells labelled at E13 (square), E15 (triangle) and E17 (circle) are shown along the respiratory trees. The three portions (I, II and III) in the mature (P21) airways ( a ) are illustrated on the schematics of the E19 lung. ( c ) Percentage of labelled cells at indicated positions (I, II and III) relative to those in the extrapulmonary bronchus of the same lung that have been lineage-labelled at E13 (square), E15 (triangle) and E17 (circle). H: high (67–100%), M: medium (33–67%), L: low (0–33%). ( d ) Stereomicroscope images of a whole-mount immunostained P21 lung lineage-labelled at E17. The conducting airways are traced with white dashed lines, and the BADJs at the front and back of the branch are marked with solid and dashed red lines, respectively. The lineage-labelled cells at the BADJ are marked with horizontal carets. Scale: 20 μm. Full size image Therefore, a second wave of conducting airway differentiation marked by SOX2 expression, follows, but terminates earlier than, the first wave to establish the BADJs ( Fig. 3b ). From the viewpoint of branching morphogenesis, the non-branching epithelium left behind by the first wave becomes SOX2-positive conducting airways early in development but becomes SOX2-negative alveolar cells late in development—a temporal switch in cell fate that sets the BADJ. Role of candidate morphogens in the two waves We reasoned that if a spatial signal such as a morphogen gradient specifies the BADJ in the developing lung, the morphogen may originate in either a proximal or distal location and decrease gradually along the proximal–distal axis ( Supplementary Fig. 4a,b ). Although a morphogen produced distally, such as Fgf10 (ref. 1 ), may limit the progression of the SOX2 wave early in development. However, it is not obvious why the SOX2 wave stops at E17, and does not keep following the continuous progression of the first wave and the putative distal morphogen gradient after E17 ( Supplementary Fig. 4a ). Alternatively, similar to Bicoid in the Drosophila embryo [13] , a morphogen produced proximally can promote SOX2 expression (the second wave) and fall below a functional threshold at the BADJ as the respiratory tree grows during development—a model likely depending on precise regulation of branch size and generation ( Supplementary Fig. 4b ). We first examined the roles of candidate morphogens in the Fgf , Wnt and Bmp signalling pathways in the progression of the two developmental waves and the formation of the BADJ. To distinguish their roles in the progression versus termination of the SOX2 wave, we used Sox9 CreER to specifically target early (E12–E15) or late (E15–E18) development. When we expressed a hyperactive Kras allele or deleted Ctnnb1 to alter receptor tyrosine kinase (including Fgf ) or Wnt signallings, the first wave was affected in both early and late development ( Fig. 4a ). Specifically, Kras mutant branches were overgrown with expanded SOX9 expression and Ctnnb1 mutant branches mostly lost SOX9 expression. Therefore, consistent with our conclusion that the two epithelial compartments are generated by a continuous wave of branching morphogenesis ( Fig. 2 ), Fgf and Wnt signallings regulate the first wave in a similar way in both early and late lung development. 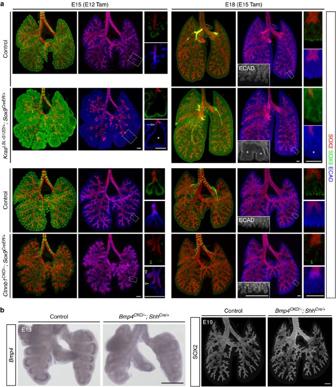Figure 4: Role of candidate morphogens in the progression of the two waves. (a) OPT images of whole-mount immunostained E15 (left panels) and E18 (right panels) lungs from littermate embryos that have been injected with tamoxifen (Tam) at E12 and E15, respectively. The boxed regions are shown as a section view for E15 and as a projection view for E18. Stereomicroscope images are shown as insets for ECAD staining at E18 for higher resolution. The accessory lobes of E18Kraslungs are removed for clarity. The first (SOX9) wave is affected similarly at both time points, including formation of overgrown branches (asterisk) with expanded SOX9 expression in theKrasmutant and loss of SOX9 expression (open green arrowhead) in theCtnnb1mutant. The second (SOX2) wave is affected at E15 when its progression has been coupled with the first wave, including a restricted (open arrow) or expanded (open arrowhead, also limited SOX2-negative ECAD region in the E15 whole-lung image) SOX2 expression domain in theKrasorCtnnb1mutants, respectively. At least two independent experiments for each time point are performed with similar results. Scale: 200 μm. (b)In situhybridization (left panels) and OPT images (right panels) of whole-mount lungs from littermate embryos. Scale: 400 μm. Figure 4: Role of candidate morphogens in the progression of the two waves. ( a ) OPT images of whole-mount immunostained E15 (left panels) and E18 (right panels) lungs from littermate embryos that have been injected with tamoxifen (Tam) at E12 and E15, respectively. The boxed regions are shown as a section view for E15 and as a projection view for E18. Stereomicroscope images are shown as insets for ECAD staining at E18 for higher resolution. The accessory lobes of E18 Kras lungs are removed for clarity. The first (SOX9) wave is affected similarly at both time points, including formation of overgrown branches (asterisk) with expanded SOX9 expression in the Kras mutant and loss of SOX9 expression (open green arrowhead) in the Ctnnb1 mutant. The second (SOX2) wave is affected at E15 when its progression has been coupled with the first wave, including a restricted (open arrow) or expanded (open arrowhead, also limited SOX2-negative ECAD region in the E15 whole-lung image) SOX2 expression domain in the Kras or Ctnnb1 mutants, respectively. At least two independent experiments for each time point are performed with similar results. Scale: 200 μm. ( b ) In situ hybridization (left panels) and OPT images (right panels) of whole-mount lungs from littermate embryos. Scale: 400 μm. Full size image In contrast, the effects of early versus late gene targeting on the SOX2 wave were different. While early targeting of the Kras / Fgf or Ctnnb1 / Wnt signalling led to a restricted or expanded SOX2 expression domain, respectively, late targeting had little or no effect on SOX2 expression ( Fig. 4a ). This temporal difference suggested that the role of Fgf and Wnt signallings in proximal–distal patterning is restricted to early development when the two waves are coupled and that other mechanisms uncouple the two waves to form the BADJ. Although Bmp4 has been implicated in proximal–distal patterning of the developing lung [30] , [31] , epithelial deletion of Bmp4 had no apparent effects in either the first or second wave ( Fig. 4b ) and the resulting Bmp4 mutant mice were viable. We note that deletion of Bmp receptors disrupts lung specification and branching, suggesting involvement of additional BMP ligands [32] . Taken together, these data indicated that alterations of some distal morphogens ( Supplementary Fig. 4a ) do not affect termination of the SOX2 wave and BADJ formation. BADJ formation is independent of branch size and generation Next, we used two different genetic conditions to alter branch number, size and generation, all of which were expected to cause major structural changes and alter the slopes and/or ranges of potential morphogen gradients. Under the first condition, lung development was allowed to initiate normally up to E13, and then an Sftpc-rtTA and tetO-DTA system was used to achieve lung epithelium-specific, doxycycline-dependent cell ablation ( Fig. 5a and Supplementary Fig. 5a,b ). We found that epithelial cell ablation disrupted the branching morphogenesis wave and generated fewer and dilated branches. Under the second condition, we examined lung development in an organ size mutant ( Igf1r −/− ). We found that the Igf1r mutant lung initiated and developed normally up to E13, after which the branching morphogenesis wave progressed much more slowly and generated a smaller lung with fewer, albeit normal looking branches ( Fig. 5b and Supplementary Fig. 5c ). Under the two genetic conditions, despite opposite changes in the level or distribution of known morphogens including Fgf10 , Bmp4 and Wnt2 ( Supplementary Fig. 5d ), the SOX2 wave continued to progress behind the SOX9 wave and terminated on schedule ( Fig. 5 ). Furthermore, under both conditions, cells in the conducting airways (Clara cells, ciliated cells and neuroendocrine cells) and the gas exchange region (alveolar type I and type II cells) underwent normal differentiation ( Supplementary Fig. 5e,f ). These data suggested a robust mechanism of BADJ formation independent of counting branches or branch generations or a specific spatial signal such as a morphogen gradient that depends on precise spatial organization of the epithelial tree ( Supplementary Fig. 4a,b ). 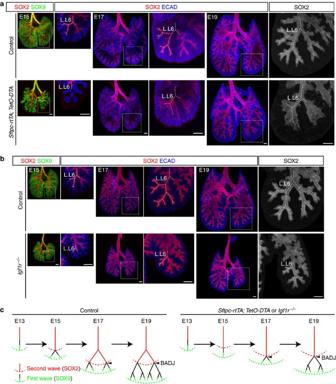Figure 5: BADJ formation is independent of branch size and generation. (a,b) OPT images of whole-mount immunostained lungs fromSftpc-rtTA; TetO-DTA(treated with doxycycline from E13 to E14) orIgf1r−/−mutant and their respective littermate control embryos. The L.L6 branch lineages14in the boxed areas are enlarged and traced with dashed lines in subsequent images. At least two experiments for each time point are performed with similar results. As illustrated in the diagram (c), in theSftpc-rtTA; TetO-DTAandIgf1r−/−mutant lungs, the first wave is still marked by SOX9 expression but progresses much slower than that in the control lungs, and the second wave follows the first wave early in development and terminates on schedule at E17. Figure 5: BADJ formation is independent of branch size and generation. ( a , b ) OPT images of whole-mount immunostained lungs from Sftpc-rtTA; TetO-DTA (treated with doxycycline from E13 to E14) or Igf1r −/− mutant and their respective littermate control embryos. The L.L6 branch lineages [14] in the boxed areas are enlarged and traced with dashed lines in subsequent images. At least two experiments for each time point are performed with similar results. As illustrated in the diagram ( c ), in the Sftpc-rtTA; TetO-DTA and Igf1r −/− mutant lungs, the first wave is still marked by SOX9 expression but progresses much slower than that in the control lungs, and the second wave follows the first wave early in development and terminates on schedule at E17. Full size image A temporal glucocorticoid signal specifies BADJ location The kinetics of the progression and termination of the SOX2 wave and its resistance to spatial perturbations prompted us to search for a temporal signal that specifies the location of the BADJ. Glucocorticoid signalling was an intriguing candidate because the level of glucocorticoid increases at late gestation stages [33] , [34] , [35] , and we found that normal BADJ formation coincided temporally with an increase in glucocorticoid signalling, as measured by plasma glucocorticoid levels and nuclear localization [36] of glucocorticoid receptor (GR) ( Supplementary Fig. 6a,b ). To test the role of glucocorticoid and other hormones, we established an explant culture assay using lungs from genetically engineered mice that allowed us to monitor the progression of the two waves in real time ( Fig. 6a ). Using this assay, we tested agonists and antagonists of glucocorticoid and other hormones, including retinoic acid and thyroid hormone, that have been implicated in lung development [37] , [38] , [39] , [40] . Whereas pharmacological alterations of other hormones had no effect or nonspecific toxicity on the cultured lungs, addition of 100 nM dexamethasone, an agonist of glucocorticoid signalling ( Supplementary Fig. 5c ), specifically terminated progression of the second wave without affecting the first wave of branching morphogenesis ( Fig. 6a ). Microarray expression profiling and immunostaining ( Supplementary Fig. 5d,e and Supplementary Data 1 ) showed that dexamethasone prematurely activated genes associated with alveolar cell differentiation ( Sftpb , Napsa , Ctsh , Ass1 , Scnn1a , Hopx , RAGE and AQP1) within 1 and 2 days of culture. Notably, alveolar differentiation occurred immediately beyond the distal boundary of the SOX2 expression domain, consistent with premature BADJ formation in a more proximal location. The effects of dexamethasone on both progression of the SOX2 wave and alveolar differentiation were blocked by mifepristone, an antagonist of glucocorticoid signalling ( Supplementary Fig. 5e,f ). 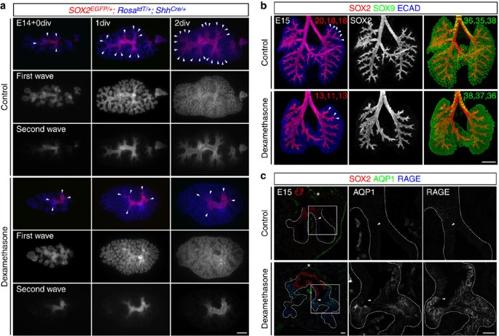Figure 6: Premature activation of glucocorticoid signalling causes a proximal shift in BADJ location in culture andin vivo. (a) Stereomicroscope images of lung slices from an E14Sox2EGFP/+; RosatdT/+; ShhCre/+embryo at the beginning of the culture (E14+0 div) or cultured for 1 (1 div) or 2 (2 div) days in the absence (Control) or presence (Dexamethasone) of dexamethasone. Arrowheads indicate the distal boundary of theSox2EGFPexpression domain. To keep a consistent colour scheme, the green fluorescence fromSox2EGFP/+and the red fluorescence fromRosatdT/+; ShhCre/+are pseudo-coloured red and blue, respectively. div, daysin vitro. Scale: 200 μm. (b,c) OPT images of E15 whole-mount immunostained lungs (b, scale: 500 μm) and confocal images of E15 immunostained lung sections (c, scale: 20 μm) from control embryos or embryos treated with dexamethasone in drinking water from E12in vivo. Arrowheads indicate the distal boundary of the SOX2 expression domain. The numbers of SOX2-positive termini (red number,P=0.002, Student’st-test) or SOX9-positive (green number,P=0.56, Student’st-test) tips from three lungs (the first number corresponding to the lung shown) are quantified. The epithelia are traced with dashed lines and the boxed areas are enlarged in subsequent images. There is a very low level of RAGE expression and no AQP1 expression in the control epithelium. Asterisks indicate normal expression of AQP1 in the vasculature. The teratogenic effects of dexamethasone limit the extent of signalling activationin vivoand restrict the sizes of the embryo and the lung. Figure 6: Premature activation of glucocorticoid signalling causes a proximal shift in BADJ location in culture and in vivo . ( a ) Stereomicroscope images of lung slices from an E14 Sox2 EGFP/+ ; Rosa tdT/+ ; Shh Cre/+ embryo at the beginning of the culture (E14+0 div) or cultured for 1 (1 div) or 2 (2 div) days in the absence (Control) or presence (Dexamethasone) of dexamethasone. Arrowheads indicate the distal boundary of the Sox2 EGFP expression domain. To keep a consistent colour scheme, the green fluorescence from Sox2 EGFP/+ and the red fluorescence from Rosa tdT/+ ; Shh Cre/+ are pseudo-coloured red and blue, respectively. div, days in vitro . Scale: 200 μm. ( b , c ) OPT images of E15 whole-mount immunostained lungs ( b , scale: 500 μm) and confocal images of E15 immunostained lung sections ( c , scale: 20 μm) from control embryos or embryos treated with dexamethasone in drinking water from E12 in vivo . Arrowheads indicate the distal boundary of the SOX2 expression domain. The numbers of SOX2-positive termini (red number, P =0.002, Student’s t -test) or SOX9-positive (green number, P =0.56, Student’s t -test) tips from three lungs (the first number corresponding to the lung shown) are quantified. The epithelia are traced with dashed lines and the boxed areas are enlarged in subsequent images. There is a very low level of RAGE expression and no AQP1 expression in the control epithelium. Asterisks indicate normal expression of AQP1 in the vasculature. The teratogenic effects of dexamethasone limit the extent of signalling activation in vivo and restrict the sizes of the embryo and the lung. Full size image Similarly, when administered in vivo to pregnant mice before BADJ formation, dexamethasone also caused a significant delay in progression of the second wave without affecting the first wave ( Fig. 6b ). Importantly, the dexamethasone-treated lungs prematurely activated expression of alveolar cell markers (RAGE and AQP1, Supplementary Fig. 7a,b ) immediately beyond the distal boundary of the SOX2 expression domain, and therefore formed the BADJ at a more proximal location of the epithelial tree ( Fig. 6c ). The location of cells undergoing premature alveolar differentiation both in culture and in vivo suggested that SOX2-negative cells, but not committed SOX2-positive conducting airway cells, are able to respond to systemic glucocorticoid signalling and differentiate into alveolar cells. The fact that cells normally destined to adopt the conducting airway fate switched to the alveolus fate in response to dexamethasone showed that the cell fate choice between the two compartments, and therefore BADJ location, is determined not by the first wave but rather the termination of the second wave in response to glucocorticoid signalling. Therefore, when there is a change in the timing of the hormonal signal, there is a corresponding change in the BADJ location. Conversely, in GR mutants ( GR −/− ) in which glucocorticoid signalling is abolished, the second wave was prolonged resulting in an expanded conducting airway compartment and a distal shift of the BADJ location ( Fig. 7a ). Although the second wave eventually stopped at E19, suggesting the existence of late-acting back-up signals other than glucocorticoids, the formation of the BADJs was not complete because the expression levels of alveolar cell markers (RAGE and AQP1) were lower than those in the control ( Supplementary Fig. 7c–e ). Interestingly, the GR mutant lung had larger SOX9-positive branch tips than the control lung ( Fig. 7b ), suggesting that glucocorticoid signalling promotes alveolar differentiation and limits both conducting airway differentiation and SOX9-positive progenitor maintenance. A proliferation marker CCND1 (Cyclin D1) was highly expressed in distal SOX9-positive and proximal SOX2-positive cells, but at a much lower level in differentiated alveolar cells in between ( Fig. 7b ), supporting the idea that BADJ formation is associated with cell cycle exit and alveolar differentiation of SOX2-negative cells left behind by the first SOX9 wave. 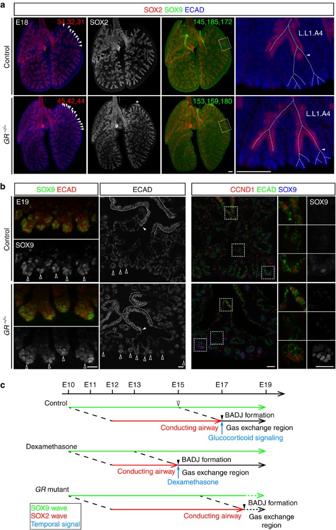Figure 7: Loss of glucocorticoid activity causes a distal shift in BADJ location. (a) OPT images of whole-mount immunostained lungs. Arrowhead, distal boundary of the SOX2 expression domain. The numbers of SOX2-positive termini (red number,P=0.0008, Student’st-test) or SOX9-positive (green number,P=0.8, Student’st-test) tips from three lungs (the first number corresponding to the lung shown) are quantified. The L.L1.A4 branch lineages14in the boxed areas are enlarged and traced with dashed lines in subsequent images. The accessory lobes are removed for clarity. The asterisk indicates blood autofluorescence. Scale: 500 μm. (b) Confocal images of immunostained lungs. CCND1, Cyclin D1. Left panels: white lines, conducting airways; filled arrowheads, BADJs; open arrowheads, branch tips. TheGRmutant has larger SOX9-positive branch tips shown in a stack projection view on the left and as a result has more recognizable branch tips on a section view on the right. Right panels: the boxed areas are enlarged in subsequent images. Note that non-epithelial cells also express CCND1. Scale: 20 μm. (c) Diagrams illustrating that BADJ formation is specified by a temporal mechanism. The first wave of branching morphogenesis (the SOX9 wave) persists throughout embryonic development (green arrow). The second wave of conducting airway differentiation (the SOX2 wave) follows the first wave, prospectively marks the conducting airways and terminates at E17 (red arrow), after which the differentiation of gas exchange region begins (black arrow). Cells near the BADJ are generated at E15 by the SOX9 wave (open arrowhead) and the BADJ forms at E17 after the SOX2 wave terminates (closed arrowhead). Long dashed lines connecting the two waves show the temporal delay between branch generation and SOX2 expression. A low level of SOX2 expression is present in part of the main bronchi at E11. An increase in glucocorticoid signalling (light blue arrow) coincides temporally with BADJ formation and premature activation of glucocorticoid signalling (dexamethasone) terminates the second wave early and causes a proximal shift in BADJ location. Loss of GR prolongs the second wave and causes a distal shift in BADJ location associated with defects in alveolar differentiation (dashed black arrow) and SOX9-positive progenitor cell maintenance (green dashed arrow). Figure 7: Loss of glucocorticoid activity causes a distal shift in BADJ location. ( a ) OPT images of whole-mount immunostained lungs. Arrowhead, distal boundary of the SOX2 expression domain. The numbers of SOX2-positive termini (red number, P =0.0008, Student’s t -test) or SOX9-positive (green number, P =0.8, Student’s t -test) tips from three lungs (the first number corresponding to the lung shown) are quantified. The L.L1.A4 branch lineages [14] in the boxed areas are enlarged and traced with dashed lines in subsequent images. The accessory lobes are removed for clarity. The asterisk indicates blood autofluorescence. Scale: 500 μm. ( b ) Confocal images of immunostained lungs. CCND1, Cyclin D1. Left panels: white lines, conducting airways; filled arrowheads, BADJs; open arrowheads, branch tips. The GR mutant has larger SOX9-positive branch tips shown in a stack projection view on the left and as a result has more recognizable branch tips on a section view on the right. Right panels: the boxed areas are enlarged in subsequent images. Note that non-epithelial cells also express CCND1. Scale: 20 μm. ( c ) Diagrams illustrating that BADJ formation is specified by a temporal mechanism. The first wave of branching morphogenesis (the SOX9 wave) persists throughout embryonic development (green arrow). The second wave of conducting airway differentiation (the SOX2 wave) follows the first wave, prospectively marks the conducting airways and terminates at E17 (red arrow), after which the differentiation of gas exchange region begins (black arrow). Cells near the BADJ are generated at E15 by the SOX9 wave (open arrowhead) and the BADJ forms at E17 after the SOX2 wave terminates (closed arrowhead). Long dashed lines connecting the two waves show the temporal delay between branch generation and SOX2 expression. A low level of SOX2 expression is present in part of the main bronchi at E11. An increase in glucocorticoid signalling (light blue arrow) coincides temporally with BADJ formation and premature activation of glucocorticoid signalling (dexamethasone) terminates the second wave early and causes a proximal shift in BADJ location. Loss of GR prolongs the second wave and causes a distal shift in BADJ location associated with defects in alveolar differentiation (dashed black arrow) and SOX9-positive progenitor cell maintenance (green dashed arrow). Full size image Finally, to examine the direct target cells of glucocorticoid signalling, we genetically deleted GR in either epithelial cells or a majority of mesenchymal cells with Shh Cre or Dermo1 Cre , respectively ( Supplementary Fig. 8a ). Mesenchymal deletion of GR partially recapitulated the expanded conducting airway compartment phenotype of the GR null mice ( Supplementary Fig. 8b ), suggesting compensation by the remaining GR-positive mesenchymal cells and/or cooperation of glucocorticoid signallings in both epithelial and mesenchymal cells [41] , [42] , [43] , [44] . Taken together, we conclude that the BADJ is specified by two nested developmental waves under the control of a temporal glucocorticoid signal ( Fig. 7c ). The results support a novel model of compartment boundary formation in the mouse lung: a first wave generates both compartments; a second wave follows the first wave to specify one compartment; and a temporal hormonal signal terminates the second wave to set the compartment boundary. Compartment boundaries including the BADJ are spatial landmarks; their formation is fundamentally the specification of different cell types on the opposite sides of the boundary and their location is often encoded spatially, for example, by morphogen gradients. However, we show that BADJ formation is because of a temporal switch in cell fate specification—the non-branching epithelia left behind by the first wave undergo conducting airway differentiation early in development, but alveolar differentiation late in development, and that the location of the BADJ is encoded temporally—by the timing of a global hormonal signal. Although glucocorticoid signalling is known to promote alveolar differentiation, our study demonstrates its new role in spatial patterning. Our results suggest that the pro-alveolus action of glucocorticoid signalling depends on the absence of SOX2 expression and in part involves mesenchyme-derived soluble [43] and/or matrix proteins [41] , [44] . How these factors impinge on cell cycle exit and alveolar differentiation requires further investigation. This time-controlled two-wave model has some unique properties in controlling compartment boundary formation in a complex organ. For example, a global temporal signal bypasses the challenges in maintaining a stable morphogen gradient at a time when the shape and size of an organ are highly dynamic and allows synchronized formation of hundreds of boundaries between two compartments, such as the BADJs. Moreover, our model contains modular programmes that are simpler to encode genetically and to modulate during evolution. For example, to evolve different numbers of branches to match respiratory demand, different species need only adjust the rate of branch generation in the first wave, while the coupling between the timing of the temporal signal and the gestation period, as well as between the respiratory and vascular trees, will ensure a functional and properly proportioned lung at birth. We suggest that, in a structure where one compartment is built upon and therefore after a previously formed compartment, such as the two epithelial compartments of the mammalian lung and vertebrate somites [12] , temporal signals may be used in addition to spatial signals or morphogen gradients to specify compartment boundaries. Our model does not exclude the role of morphogens, including Fgf , Wnt and Bmp , in the first wave and in the coupling of the two waves in early lung development. In fact, the same signalling pathways (for example, Fgf and Wnt ) are continuously required for the first wave throughout embryonic development. However, the BADJ forms in late lung development apparently independent of these morphogens, but rather in response to a temporal signal. Different from the multipotent progenitor model [15] , our model indicates that early and late progenitors share the same branching programme and the capability of responding to glucocorticoids, and only start to differ when they become branch stalks and undergo differentiation in response to a global hormonal signal. Our model also suggests that the BASCs are the last cells committed to the conducting airway cell fate when the glucocorticoid signal is activated. Such a developmental history might endow the BASCs the abilities to possibly generate cells of both epithelial compartments under certain injury conditions [7] , [45] , [46] . Our findings that branching morphogenesis continues throughout development and generates branches for both epithelial compartments provide new insights into proximal–distal patterning in the lung. Although the spatial distributions of SOX9 and SOX2 have been described in the early developing lung with SOX9 expressed in the distal branching epithelia and SOX2 expressed in the proximal non-branching epithelia [1] , this proximal–distal patterning does not simply extend to the late developing lung (after E17). We show that branching morphogenesis continues during late development and leaves behind non-branching epithelia wrapped by smooth muscles and co-aligned with vessels, similar to the proximal non-branching epithelia during early development. These late non-branching epithelia are proximal relative to the distal SOX9 wave, but do not express SOX2 as the early non-branching epithelia do and instead differentiate into alveolar cells. Therefore, the proximal non-branching portion of the respiratory tree in late lung development can be further divided into two parts: SOX2-positive conducting airways most proximally and SOX2-negative alveolar cells in the near distal region. Additional mechanism other than SOX2-proximal/SOX9-distal patterning is necessary to explain why the near distal, non-branching epithelia during late lung development do not activate SOX2. We show that such a mechanism involves a temporal glucocorticoid signalling that terminates the SOX2 wave and sets the BADJ. Our two-wave model is also supported by and predicts the existence of the alveolar duct—a tubular structure distal to the BADJ made of alveolar cells, which is derived from branches left behind by the first wave during late lung development and undergoing alveolar differentiation in response to the hormonal signal. Our model suggests mechanism-based therapeutic options for lung defects in premature birth. As the first wave of branching morphogenesis progresses throughout embryonic development, lungs in premature infants will have structural immaturity, such as fewer branches for the gas exchange compartment, in addition to cellular immaturity, such as insufficient surfactant production [47] . Since cells at the front of the first wave express the same molecules and signalling genes throughout development, positive and negative regulators of branching in early lung development may also be therapeutic targets for accelerating the branching morphogenesis wave in the perinatal period to compensate for the shorter developmental time in premature births. Although the conducting airways and gas exchange region in the mature lung are distinct compartments separated by the BADJ, their embryonic precursors are surprisingly plastic such that the location of the BADJ can be altered simply by manipulating the timing of the glucocorticoid signal. Such plasticity suggests that the beneficial effect of glucocorticoid therapy in premature birth [48] , [49] is at least in part through its effect on BADJ position and balancing the proportion of the two compartments. Mice Inbred FVB/NJ (Stock 001800) and C57B6/J (Stock 000664) were obtained from the Jackson Laboratory. Mice carrying Sox9 CreER (ref. 50 ), Kras LSL-G12D (ref. 51 ), Sox2 CreER (ref. 52 ), Rosa mTmG (ref. 53 ), Sox2 EGFP (ref. 52 ), Sftpc-rtTA (ref. 54 ), TetO-DTA (ref. 55 ), TetO-GFP (ref. 56 ), Rosa tdT (ref. 57 ), Shh Cre (ref. 58 ) and Dermo1 Cre (ref. 59 ) alleles have been described. Mice carrying the Igf1r (ref. 60 ), GR (ref. 61 ), Bmp4 (ref. 62 ) or Ctnnb1 (ref. 63 ) conditional allele were mated to female HPRT Cre/+ mice [64] to generate mice carrying the germline Igf1r null allele ( Igf1r − , GR − , Bmp4 − and Ctnnb1 − ). The resulting null alleles were genotyped using the following primer pairs: 5′-TGAGACGTAGCGAGATTGCTGTA-3′ and 5′-CAGGCTTGCAATGAGACATGGG-3′ ( Igf1r − ); 5′-CTCCTCCATTTTGCGAGC-3′ and 5′-AAGGAGCAGTCACCAACTGTC-3′ ( GR − ); 5′-AGACTCTTTAGTGAGCATTTTCAAC-3′ and 5′-AAGATGCCTGCCAGGACTGA-3′ ( Bmp4 − ); and 5′-CACCATGTCCTCTGTCTATTC-3′ and 5′-TACACTATTGAATCACAGGGACTT-3′ ( Ctnnb1 − ). The day the vaginal plug was observed was designated as E1 and the day the mice were born was designated as P0. For FVB/NJ and C57B6/J mice, the last day of gestation is E19. For Sox2 CreER lineage tracing experiments, 0.45 mg tamoxifen (T5648, Sigma) dissolved in corn oil (C8267, Sigma) was given orally to timed pregnant mice at indicated gestation days and the progenies were allowed to grow to P21 when the lungs were harvested. A higher dose of tamoxifen caused embryonic or neonatal death. We note that, although it takes 12–24 h to observe Cre-dependent reporter expression [65] , recombination likely occurs much earlier and is directly relevant to inferring the time of BADJ formation in the long-term Sox2 CreER lineage tracing experiments. For Sox9 CreER lineage tracing and Kras activation experiments, 2 mg tamoxifen dissolved in corn oil was given intraperitoneally to timed pregnant mice. To delete Ctnnb1 with Sox9 CreER , 3.5 mg tamoxifen dissolved in corn oil was given intraperitoneally to timed pregnant mice. To activate Sftpc-rtTA , timed pregnant mice were given 2 mg ml −1 doxycycline (D9891, Sigma) in drinking water from E13 to E14. To activate glucocorticoid signalling, timed pregnant mice were given 0.5 μg ml −1 dexamethasone (D2915, Sigma) in drinking water from E12 to E15. At least three independent dexamethasone treatments were carried out with similar results. To measure plasma corticosterone levels, mice were killed with carbon dioxide around noon, blood collected in syringes containing 100 μl 0.5 M EDTA (ethylenediaminetetraacetic acid, E9884, Sigma) through inferior vena cava to minimize haemolysis and corticosterone level measured using an enzyme immunoassay kit (500655, Cayman). All animal experiments were approved by the institutional animal care and use committee (IACUC) at Texas A&M Health Science Center Institute of Biosciences and Technology (protocol number 11004). Antibodies The following antibodies were used: mouse anti-Acetylated tubulin (AcT, 1:2,500, T7451, Sigma), rabbit anti-aquaporin 1 (AQP1, 1:1,000, AB2219, Millipore), rabbit anti-CCSP (1:1,000, WRAB-3950, Seven Hills Bioreagents), goat anti-CCSP (1:2,500, Dr Barry Stripp, Duke University), rabbit anti-calcitonin gene-related peptide (1:500, BML-CA1134, Enzo Life Sciences), rabbit anti-CCND1 (1:500, RM9104S0, ThermoFisher), rabbit anti-fibroblast growth factor receptor 2 (1:250, sc-122, Santa Cruz Biotechnology), mouse anti-forkhead box protein J1 (1:100, Dr Steven Brody, Washington University in St Louis), chicken anti-green-fluorescent protein (GFP, 1:1,000, AB13970, Abcam), rat anti-ECAD (1:1,000, 131900, Invitrogen), rabbit anti-GR (1:500, sc-1004, Santa Cruz Biotechnology), hamster anti-glycoprotein 38 (1:250, 8.1.1, Developmental Studies Hybridoma Bank), rat anti-CD31 (PECAM, 1:500, 550274, BD Biosciences), rabbit anti-phospho-ERK1/2 (1:250, 4370, Cell Signaling Technology), rat anti-RAGE (1:1,000, MAB1179, R&D Systems), Cy3 or fluorescein isothiocyanate-conjugated mouse anti-SMA (1:1,000, C6198 or F3777, Sigma), goat anti-SRY-box-containing gene 2 (1:250, sc-17320, Santa Cruz Biotechnology), rabbit anti-SRY-box-containing gene 9 (1:1,000, AB5535, Millipore), goat anti-SRY-box-containing gene 9 (SOX9, 1:1,000, AF3075, R&D Systems), rabbit anti-prosurfactant protein C (SFTPC, 1:1,000, AB3768, Millipore). The goat anti-CCSP antibody, but not the rabbit anti-CCSP antibody, was sensitive enough to label the BASCs under current experimental conditions. As the SOX2 antibody was also made in goat, GFP expression in the Sox2 CreER/+ ; Rosa mTmG/+ and Sox2 EGFP/+ mice was used as a surrogate marker of SOX2 for co-labelling with the goat anti-CCSP antibody ( Supplementary Fig. 1g ). The arteries were distinguished from the veins based on their narrow lumen, association with a high density of smooth muscles, proximity to the airway and connection with the left/right main pulmonary arteries. Fluorescent donkey secondary antibodies were from Invitrogen and Jackson ImmunoResearch and were used at 1:1,000 dilution. As there was no donkey anti-hamster secondary antibodies, rabbit or goat secondary antibodies were used for the GP38 antibody ( Supplementary Fig. 1e ). Tissue preparation and immunostaining Three- to four-week-old male and female mice were anaesthetized with Avertin (T48402, Sigma) and perfused with phosphate-buffered saline (PBS, pH 7.4) through the right ventricle. Lungs were inflated with 0.5% paraformaldehyde (PFA; P6148, Sigma) in PBS at 25-cm H 2 O pressure, and then dissected and fixed with 0.5% PFA in PBS at room temperature for 3–6 h. Embryos were dissected from timed pregnant mice and fixed with 0.5% PFA in PBS at room temperature for 2–4 h. For section immunostaining, the fixed lungs were cryoprotected in PBS with 20% sucrose and 33% optimal cutting temperature compound (OCT; 4583, Tissue-Tek, Tokyo, Japan, optional for embryonic lungs) at 4 °C overnight and then embedded in OCT. Immunostaining of frozen sections and whole lungs was carried out essentially as described [66] . Briefly, frozen sections at 10-μm thickness were incubated with PBS with 5% normal donkey serum (017-000-121, Jackson ImmunoResearch) and 0.3% Triton X-100 and then incubated with primary antibodies diluted in PBS with 0.3% Triton X-100 at 4 °C overnight. The following day, the sections were washed with PBS for 2 h at room temperature and then incubated with secondary antibodies and 4′,6-diamidino-2-phenylindole (DAPI) diluted in PBS with 0.1% Triton X-100 and 0.1% Tween-20 for 90 min at room temperature. The sections were then washed as described above and mounted with Aquamount mounting medium (18606, Polysciences). The Forkhead box protein J1 antibody required an antigen-retrieval procedure before staining, in which sections were heated in sodium citrate buffer (10 mM sodium citrate, 0.05% Tween-20, pH 6.0) at 95 °C for 30 min and allowed to cool down at room temperature for an additional 30 min. For whole-mount immunostaining, the lungs were dehydrated through a methanol/PBS gradient and bleached with 6% hydrogen peroxide in methanol at 4 °C overnight. The bleached lungs were rehydrated through a methanol/PBS gradient and incubated with PBS with 5% normal donkey serum and 0.3% Triton X-100 and then incubated with primary antibodies diluted in PBS with 0.3% Triton X-100 at 4 °C overnight. The following day, the lungs were washed in PBS with 1% Triton X-100 and 1% Tween-20 for 6 h at room temperature and then incubated with secondary antibodies diluted in PBS with 0.3% Triton X-100 at 4 °C overnight. The lungs were then washed again and fixed with 4% PFA in PBS at room temperature for 2–4 h. For imaging with a fluorescence stereomicroscope, the lungs were dehydrated through a methanol/PBS gradient, cleared with BABB—one part of benzyl alcohol (24122, Sigma) and two parts of benzyl benzoate (B6630, Sigma)—and mounted on a depression well slide without a coverslip and with a minimal amount of BABB that was enough to cover the lungs. Images were captured on a fluorescence stereomicroscope with a × 2 Plan Apochromat objective (M205C, Leica) or a confocal microscope (FV1000, Olympus). OPT microscopy Immunostained whole-mount lungs were embedded in 1% low melting agarose (16520-100, Invitrogen), processed and imaged on a Bioptonics 3001 OPT scanner equipped with GFP3, TXR and Cy5 filters (Bioptonics, UK) at a high resolution (1,024 pixels) following the manufacturer’s instructions. The resulting image stacks were visualized using maximal intensity projection with the Bioptonics Viewer (Bioptonics, UK) or the Imaris (Bitplane) software. After the scan, some lung samples were dissected from the agarose block and imaged under a fluorescence stereomicroscope (M205C, Leica). Quantification of branch tips/termini and cell numbers All branches of planar bifurcation in the L.L1 through L.L6 branch lineages [14] were counted and these branches were close to the flat edge of the left lobe ( Supplementary Fig. 9 ). By combining multiple branch lineages, this branch counting method was robust to account for variations in the branch lineage that might occur as a result of space competition from neighbouring branches [67] , as well as the non-dichotomous nature of branching in the mouse lung [14] . As branches generated at early gestation stages (before E15) gradually activated Sox2 and had a high level of SOX2 expression proximally and a low level distally, only branch termini with a high-level SOX2 expression were counted. SOX9- and SOX2-expressing branches were close- and open-ended and referred to as branch tips and termini, respectively. At least three lungs were quantified for each embryonic or postnatal stage examined. For Sox2 CreER lineage tracing experiments, the conducting airways along the RCr.L1 lineage [14] of P21 lineage-labelled lungs were divided into three regions of equal length and four random fields were imaged for each region. To normalize labelling efficiency between mice, the density of GFP-positive cells in each region was compared with that in the extrapulmonary bronchus in the same lung and categorized as high (67–100%), medium (33–67%) or low (0–33%). Owing to limited resolution in whole-mount imaging, which was necessary to map the labelled cells on the respiratory tree, precise cell counting was not feasible. At least two independent lineage-labelling experiments with similar results were performed for each embryonic stage examined. Section and whole-mount in situ hybridization In situ hybridization was performed essentially as described [68] . Digoxigenin-labelled riboprobes (11277073910, Roche) were transcribed with T7 RNA polymerase (18033-019, Invitrogen) from the indicated cDNAs, which were isolated as cloned PCR products derived from mouse embryonic lung RNAs. Embryonic lungs were dissected and fixed in 4% PFA in PBS for 3–5 h at room temperature. For section in situ hybridization, fixed lungs were cryoprotected in PBS with 20% sucrose and 0.4% PFA at 4 °C overnight and then embedded in OCT. At room temperature, frozen sections at 10-μm thickness were fixed with 4% PFA in PBS for 10 min and then treated with freshly made acetylation solution (diethylpyrocarbonate-treated H 2 O with 0.0133% triethanolamine and 0.0025% acetic anhydride) for 10 min. After incubation with hybridization solution (50% formamide, 5 × SSC (sodium chloride and sodium citrate), 5 × Denhardt’s solution, 500 μg μl −1 salmon sperm DNA and 250 μg μl −1 yeast tRNA) for 1 h at room temperature, the sections were incubated with 1 μg ml −1 riboprobes diluted in hybridization solution in a slide oven (24100, Boekel) at 62 °C overnight. The following day, after being washed in 2 × SSC for 30 min at room temperature and 0.2 × SSC for 2 h at 65 °C, the sections were incubated with TBST (100 mM Tris, 150 mM sodium chloride, 0.1% Tween-20, pH 7.5) with 5% normal sheep serum (013-000-121, Jackson ImmunoResearch) and then with antidigoxigenin alkaline phosphatase Fab fragment (11093274910, Roche) diluted in TBST (1:1,000) at 4 °C overnight. The following day, the sections were washed with TBST for 2 h at room temperature and the alkaline phosphatase activity was detected with nitroblue tetrazolium (N6639, Sigma) and 5-bromo-4-chloro-3-indolylphosphate (B6149, Sigma). For whole-mount in situ hybridization, fixed lungs were separated into individual lobes, dehydrated and stored in 100% methanol at −20 °C. For some riboprobes, E17 lungs were sliced at 200~300-μm thickness orthogonal to the main bronchi of the left and right caudal lobes with a microscissor to increase permeability. At room temperature, the lungs were rehydrated through a methanol/DEPC-PBS (diethylpyrocarbonate-treated PBS) gradient, permeabilized with 20 μg ml −1 protease K (03115887001, Roche) in DEPC-PBS for 10 min and fixed with PBS with 0.25% glutaraldehyde and 4% PFA for 20 min. After incubation with pre-hybridization solution (50% formamide, 4 × SSC, 1 × Denhardt’s solution, 250 μg μl −1 salmon sperm DNA, 250 μg μl −1 yeast tRNA, 50 μg ml −1 heparin, 0.1% Tween-20) for 1 h at 62 °C, the sections were incubated with 1 μg ml −1 riboprobes diluted in hybridization solution (pre-hybridization solution with 10% >500 kDa dextran sulphate) in a slide oven (24100, Boekel) at 62 °C overnight. The following day, the lungs were washed in 50% formamide with 4 × SSC and 0.1% Tween-20 for 1 h at 65 °C, incubated with 100 μg ml −1 RNase A diluted in 100 mM Tris (pH 7.5) with 500 mM sodium chloride and 0.1% Tween-20 for 1 h at 37 °C and then washed in 50% formamide with 2 × SSC and 0.1% Tween-20 at 65 °C overnight. The following day, the lungs were blocked with TBST with 5% normal sheep serum and then incubated with antidigoxigenin alkaline phosphatase Fab fragment diluted in TBST at room temperature for 3 h and subsequently washed in TBST at 4 °C overnight. The following day, the alkaline phosphatase activity was detected with nitroblue tetrazolium and 5-bromo-4-chloro-3′-indolyphosphate. After the alkaline phosphatase reaction, the lungs were fixed with 4% PFA in PBS at 4 °C overnight, cleared with 75% glycerol and mounted on a depression well slide with coverslip for imaging. To minimize experimental variation, E14 and E17 lungs were embedded in the same OCT block and processed on the same section, and E14 lung lobes and E17 lung lobes or slices, and littermate control and mutant lung lobes were processed in the same tube for each riboprobe throughout the in situ experiment. Images were captured on an upright microscope (BX60, Olympus) or a stereomicroscope (M80, Leica). Lung explant culture E13 lungs or E14 lung slices of 200~300-μm thickness were isolated in ice-cold PBS and cultured on Whatman polycarbonate membranes (09-300-53, Fisher Scientific) in DMEM/F12 media (11320032, Invitrogen) with 1% fetal bovine serum (16140063, Invitrogen) and penicillin and streptomycin (15140148, Invitrogen). To activate Sftpc - rtTA , 2 μg ml −1 doxycycline was added to the culture media. To screen for hormonal regulators of BADJ formation, the following chemicals were added to the culture media: dexamethasone (100 nM, D2915, Sigma), 6-propyl-2-thiouracil (100 μM, P3755, Sigma), methimazole (50 μM, M8506, Sigma), acitretin (10 μM, 44707, Sigma) and mifepristone (3 μM, M8046, Sigma). Cultured lungs were imaged daily on a fluorescence stereomicroscope (M205C, Leica). Microarray expression profiling RNAs were extracted from E14 lungs cultured in control and dexamethasone media for 24 h using Trizol reagents (15596018, Invitrogen) and an RNeasy Mini kit (74104, Qiagen). Labelled cRNAs were generated using an Illumina TotalPrep RNA amplification kit (AMIL1791, Invitrogen) and hybridized to Illumina mouse WG-6 v2 expression beadchips (BD-201-0202, Illumina). The experiments were repeated with lungs from independent litters. The expression values from the microarrays were normalized using rank invariant normalization and analysed using the R statistical software. Accession codes: The microarray data have been deposited in Gene Expression Omnibus under accession number GSE56831 . How to cite this article: Alanis, D. M. et al. Two nested developmental waves demarcate a compartment boundary in the mouse lung. Nat. Commun. 5:3923 doi: 10.1038/ncomms4923 (2014).